Ultra-high aspect ratio high-resolution nanofabrication for hard X-ray diffractive optics Although diffractive optics have played a major role in nanoscale soft X-ray imaging, high-resolution and high-efficiency diffractive optics have largely been unavailable for hard X-rays where many scientific, technological and biomedical applications exist. This is owing to the long-standing challenge of fabricating ultra-high aspect ratio high-resolution dense nanostructures. Here we report significant progress in ultra-high aspect ratio nanofabrication of high-resolution, dense silicon nanostructures using vertical directionality controlled metal-assisted chemical etching. The resulting structures have very smooth sidewalls and can be used to pattern arbitrary features, not limited to linear or circular. We focus on the application of X-ray zone plate fabrication for high-efficiency, high-resolution diffractive optics, and demonstrate the process with linear, circular, and spiral zone plates. X-ray measurements demonstrate high efficiency in the critical outer layers. This method has broad applications including patterning for thermoelectric materials, battery anodes and sensors among others. Diffractive optics have played a major role in nanoscale X-ray imaging [1] and focusing in the soft X-ray region. X-ray microscopes capable of mapping material properties, performing tomography and probing various types of samples from computer chips to biological cells in the tens of nanometres resolution have become a powerful scientific tool. However, in the hard X-ray region where penetration lengths are much greater and thicker samples can be studied, it is more difficult to control the wavefront of X-rays with both high-efficiency and high-resolution owing to the difficulty in fabricating ultra-high aspect ratio diffractive optics [2] . The ability to fabricate high-efficiency hard X-ray diffractive optics using vertical directionality controlled metal-assisted chemical etching (V-MACE) ( Fig. 1a ) opens up new opportunities for high-resolution microscopy with compact X-ray sources and for more sophisticated wavefront manipulating capabilities for synchrotrons and X-ray-free electron lasers. 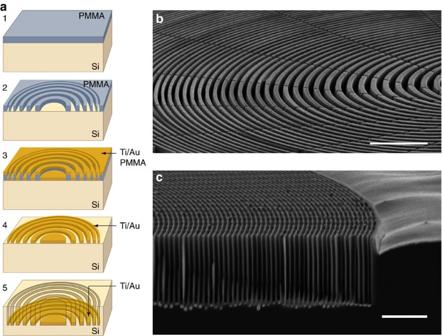Figure 1: Process flow and high aspect ratio zone plates. (a) Schematic of general process flow for metal-assisted chemical etching (MACE). (a1) Resist is spun on the wafer. (a2) Resist is exposed and developed. (a3) A thin layer of Ti and Au is electron-beam-evaporated onto the sample, and a liftoff is performed. (a4) The metal layer remains on the top of the wafer. The sample and etchant mixture consisting of HF, H2O2and H2O are cooled. (a5) A droplet of the etchant is placed onto the sample and etching takes place. The mask moves with the etching front, creating structured trenches in the silicon. Vertical directionality controlled MACE causes the etching front to proceed vertically, and in this case is controlled by the pattern design in step 2, the thickness of the metal layers in step 3, and the temperature of the etching in step 5. (b) Scanning electron microscope (SEM) image of a zone plate pattern produced using vertical directionality controlled MACE. Scale bar, 5 μm. (c) Cross-sectional view of the zone plate produced using V-MACE. The outermost zone widths of the zone plate are 100 nm. Scale bar, 2 μm. Figure 1: Process flow and high aspect ratio zone plates. ( a ) Schematic of general process flow for metal-assisted chemical etching (MACE). ( a 1) Resist is spun on the wafer. ( a 2) Resist is exposed and developed. ( a 3) A thin layer of Ti and Au is electron-beam-evaporated onto the sample, and a liftoff is performed. ( a 4) The metal layer remains on the top of the wafer. The sample and etchant mixture consisting of HF, H 2 O 2 and H 2 O are cooled. ( a 5) A droplet of the etchant is placed onto the sample and etching takes place. The mask moves with the etching front, creating structured trenches in the silicon. Vertical directionality controlled MACE causes the etching front to proceed vertically, and in this case is controlled by the pattern design in step 2, the thickness of the metal layers in step 3, and the temperature of the etching in step 5. ( b ) Scanning electron microscope (SEM) image of a zone plate pattern produced using vertical directionality controlled MACE. Scale bar, 5 μm. ( c ) Cross-sectional view of the zone plate produced using V-MACE. The outermost zone widths of the zone plate are 100 nm. Scale bar, 2 μm. Full size image High-resolution, high-efficiency X-ray diffractive optics, such as zone plates, are challenging to fabricate because of the need to make dense, very high aspect ratio, nanoscale structures to maintain both high spatial resolution and high diffraction efficiency. The smallest features, located at the outermost zones of the zone plate, define the numerical aperture of the lens at a given wavelength. The diffraction efficiency is related to the zone thicknesses, wavelength, and material. Higher X-ray energies require thicker zones for efficient focusing and, therefore, require zone plates with ultra-high aspect ratio nanostructures. For extremely high aspect ratio and high resolutions typically <10 nm, volume effects [3] , [4] , [5] occur, and to gain efficiency zones must be tilted/tapered. Current methods used to produce X-ray diffractive optics include top-down methods involving patterning of a thick resist mould [6] , [7] , pattern transfer into a substrate using deep reactive ion etching [8] , [9] , [10] , anisotropic Si wet etch [11] , [12] , multiple patterning techniques [13] , multilayer Laue lens, various multilayer-sliced zone plate techniques [14] , lithographic stacking [15] and mechanical stacking [16] . Advantages and tradeoffs exist with each method. For example, traditional top-down diffractive optics fabrication methods commonly result in aspect ratios of 12:1 or less, but are relatively simple to produce. Mechanical stacking is currently the most used technique for producing high aspect ratio X-ray diffractive optics. Although possible, challenges exist for stacking more than two zone plates. Multilayer Laue lenses can achieve very high aspect ratio but are limited to linear structures and small effective areas. Focusing in two dimensions requires a pair of lenses and a reduction in efficiency proportional to the number of lenses used. Multilayer-sliced zone plate techniques such as the method using atomic layer deposition and focused ion beam can produce very high aspect ratio structures with very small feature sizes but are limited to circular structures, small effective areas and errors in zone shapes. The benefits of fabricating diffractive X-ray optics using the technique described here include the ability to fabricate large area structures, important for maintaining sufficient working distance, with arbitrary geometries and patterns, the ability to focus in two dimensions using a single diffractive optical element and the simplicity of a single-step lithographic process. MACE using noble metals, first reported by Li and Bohn [17] , is a simple and low-cost method used to fabricate Si nanowires, nanoporous silicon and nanopillars [18] , [19] , [20] , [21] . Several reviews [22] , [23] can be found on the topic of MACE. In MACE, a noble metal layer, such as Au, is patterned onto the substrate. This serves as the etch mask. An etchant solution consisting of hydrogen peroxide (H 2 O 2 ), hydrofluoric acid (HF) and water (H 2 O) is placed onto the pattern and substrate, and Si is etched, creating trenches in the substrate. Movement of the metal catalyst during the etching process, such as sliding, rotation and folding [24] , has been shown to create interesting three-dimensional patterns. However, because of this movement, the aspect ratio achievable for vertical features in an isolated, arbitrary pattern has been limited. In this paper, we describe vertical directionality controlled MACE (V-MACE), a method capable of fabricating vertical features in an arbitrary nanoscale pattern with over 100:1 aspect ratio, and use it to create ultra-high aspect ratio X-ray zone plates such as those illustrated in Fig. 1b . V-MACE involves the use of additional electron-hole-concentration balancing structures, metal anchors internal or external to a desired structure and appropriate etch chemistry. Advantages of this method include the ability to etch a defined pattern specific to the application of interest including complex, curved, linear or non-linear patterns. It is also a simple fabrication method requiring only a single lithography step combined with a wet etch. Large diameter optics combined with ultra-high aspect ratio features at high resolution can be achieved, and the structure fabricated using this method is easily compatible with common metallization techniques as well as mechanical stacking methods. As a demonstration of the utility of this fabrication technique, platinum atomic layer deposition of a Si zone plate mould is described, along with zone plate efficiency measurements using 8.995 keV X-rays, which resulted in a 20.1% first-order efficiency with the highest resolution zones. Effect of electron-hole concentration balancing structures During MACE, electron holes are constantly generated and injected into silicon. They diffuse into the silicon isotropically and can be modelled as a two-dimensional constant-source diffusion process described by complementary error functions [19] . Therefore, as MACE progresses, the electron holes diffuse to the vicinity of each Au–Si interfaces, eventually, evolving to a profile distribution where the electron-hole concentration is highest at the centre of the Au metal films, gradually decreasing towards the edge. This non-uniform electron hole distribution leads to differences in etch rates throughout a structure and is evidenced in the ‘outward splaying’ effect observed in all our deep etch experiments, preventing the ability to create a vertical etch profile for isolated structures, as seen in Fig. 2a . 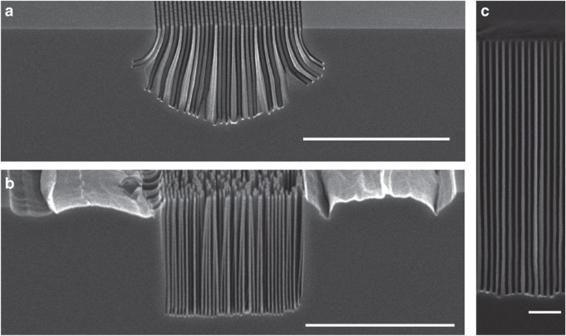Figure 2: Effect of electron-hole concentration balancing structures. (a) SEM image of an isolated array of 125 nm lines and spaces etched using MACE without vertical directionality control. Splaying results as a result of the imbalance in electron-hole concentration. Scale bar, 10 μm. (b) SEM image of an isolated array of 125 nm lines and spaces etched using MACE with vertical directionality control. Electron-hole balancing structures are shown to either side of the isolated line array. Lines are etched vertically. Scale bar, 10 μm. (c) SEM image of 100 nm 1:1 lines, 6.6 μm tall. Scale bar, 1 μm. Figure 2: Effect of electron-hole concentration balancing structures. ( a ) SEM image of an isolated array of 125 nm lines and spaces etched using MACE without vertical directionality control. Splaying results as a result of the imbalance in electron-hole concentration. Scale bar, 10 μm. ( b ) SEM image of an isolated array of 125 nm lines and spaces etched using MACE with vertical directionality control. Electron-hole balancing structures are shown to either side of the isolated line array. Lines are etched vertically. Scale bar, 10 μm. ( c ) SEM image of 100 nm 1:1 lines, 6.6 μm tall. Scale bar, 1 μm. Full size image This splaying can be corrected using electron-hole concentration balancing structures to create a more uniform electron-hole distribution so as to induce a constant etch rate and thus achieve a vertical etch profile. Balancing structures are any additional structures located in regions where there is a large electron-hole concentration difference. For example, they can be used at the edges of isolated structures that provide additional electron-holes in the silicon during the MACE, and thus balanced concentration in the vicinity of areas where vertical etch directionality is desired. Balancing structures can take the form of a variety of geometries such as a plane catalyst stripe, perforated catalyst stripe, or any other means, not limited to the use of an additional metal catalyst, of creating a balanced electron-hole concentration at the edges, for example, using localized electric currents. In addition, the balancing structure can be induced in any direction relative to the isolated feature, to the side, above or below, such that the desired electron-hole concentration balance is obtained within the region of interest, and etch rates in this region become uniform. As a demonstration of the effect of electron-hole concentration balancing structures, a high aspect ratio isolated linear grating has been fabricated, with and without the balancing structures, as seen in Fig. 2 . The linear grating is 10 μm in width with a half period of 125 nm. Figure 2a shows a cross-section of the linear grating without the use of electron-hole concentration balancing structures. A splaying of the edges of features due to electron-hole concentration differences leads to non-vertical etching. Figure 2b shows a cross-section of the linear grating with the use of hole concentration balancing structures. The balancing structures in this case are solid stripes of Au catalyst 10 μm in width surrounding the edges of the linear grating. The catalyst dimensions and shape can be tailored to result in minimal disturbance to the final device, or to be used for further processing, for example, electroplating. It can be seen that the effects of the electron-hole concentration balancing structures result in vertical etch control of the linear grating. Figure 2c demonstrates high aspect ratio fabrication of silicon gratings using this method. The grating in Fig. 2c has a half period of 100 nm and is 6.6 μm tall, resulting in an aspect ratio of 66:1. High aspect ratio zone plates We have fabricated ultra-high aspect ratio X-ray zone plates using this method. In order to obtain additional rigidity in the metal film catalyst to prevent catalyst movements such as folding and sliding, thus minimizing distortion of the metal films during the etching, we add metal anchors to the metal film catalyst. The metal anchors in this case are external to the zones so that each of the zones becomes interconnected. This is illustrated in Fig. 3a . Variations in the anchoring pattern can result in different mechanical responses of the catalyst during etching. Some variations are shown in the SEM images of zone plate portions in Fig. 3b,c . In addition, to help mitigate the collapse of the zones during drying, we add buttressing structures that are discontinuities in the metal catalyst, such that the silicon zones can also be interconnected. This is useful for helping mechanically stabilize the silicon structure during the drying process and during further processing. It is also useful for the creation of a silicon free-standing zone plate or any other interconnected silicon structure. 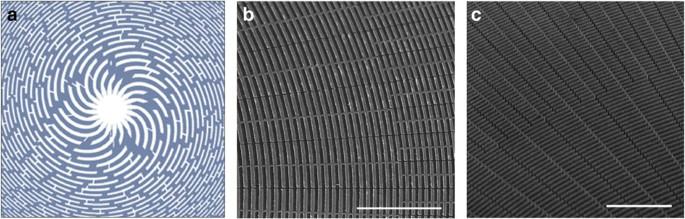Figure 3: Metal interconnections and zone plate buttresses. (a) CAD image of metal interconnections and zone plate buttresses in a spiral zone plate data set. (b,c) Representative SEM images of metallized patterns produced by liftoff showing the metal interconnections as well as the gaps, which are the buttresses of the zone plate. Scale bars, 5 μm. Figure 3: Metal interconnections and zone plate buttresses. ( a ) CAD image of metal interconnections and zone plate buttresses in a spiral zone plate data set. ( b , c ) Representative SEM images of metallized patterns produced by liftoff showing the metal interconnections as well as the gaps, which are the buttresses of the zone plate. Scale bars, 5 μm. Full size image Mechanical anchors can be external or internal to the feature. External anchors hold portions of the pattern together that, in this case, are the different zones. Internal anchors are created by holes in the catalyst that are smaller than the structure that needs to be patterned. They can be used both for stability in the metal catalyst film and as a means for etching larger features, giving a physical pathway for etchants to diffuse. The remaining structures left by the internal anchors can be removed through various techniques including silicon oxidation and HF etching. 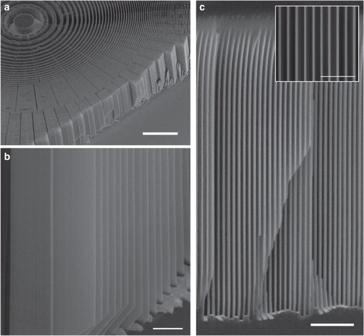Figure 4: High aspect ratio zone plates. (a) SEM image of a deeply etched zone plate with a mechanically cleaved portion showing the cross-section. Scale bar, 10 μm. (b) Side profile of the lines in cross-section. The thin lines in the centre are the zone plate buttresses providing structural stability to the consecutive zones. Metal is seen at the bottom of the zones. Sidewalls are smooth. Scale bar, 500 nm. (c) Cross-sectional image of the zones demonstrating very deep, vertical etching. Scale bar, 2 μm. The inset shows that the line widths are 51 nm at an ~1:3 line to space ratio. Scale bar in the inset, 1 μm. Figure 4a illustrates the fabrication of a very high aspect ratio zone plate in silicon with a diameter of 100 μm, outermost zone width of 100 nm and a duty cycle of 1:3. The duty cycle was designed such that atomic layer deposition can be performed later for zone doubling [13] , or so that the zone plate can be used for higher order diffraction [25] . The zone plate was mechanically cleaved to examine the cross-section. Figure 4b shows the sidewalls of this cross-section. The sidewalls after this etch are quite smooth and determined by the roughness in the metal catalyst. The thin vertical line, 30 nm in width, shown at the centre of the tilted zone segment is a silicon buttresses that connects the neighbouring zones. They can also be seen in Fig. 4a . The cross-section clearly demonstrates that high aspect ratio features with a vertical profile has been achieved. Shown in Fig. 4c are lines that have 100 nm half period and are 14 μm tall. However, porous silicon formation can be seen at the top of the structures along with some curvature. These can easily be removed with a silicon etch. The vertical portion of the features remains at over 12 μm tall, leading to an aspect ratio >120:1. The inset in Fig. 4c shows a zoomed-in version of the lines, and control of the silicon lines, at 51 nm width. Figure 4: High aspect ratio zone plates. ( a ) SEM image of a deeply etched zone plate with a mechanically cleaved portion showing the cross-section. Scale bar, 10 μm. ( b ) Side profile of the lines in cross-section. The thin lines in the centre are the zone plate buttresses providing structural stability to the consecutive zones. Metal is seen at the bottom of the zones. Sidewalls are smooth. Scale bar, 500 nm. ( c ) Cross-sectional image of the zones demonstrating very deep, vertical etching. Scale bar, 2 μm. The inset shows that the line widths are 51 nm at an ~1:3 line to space ratio. Scale bar in the inset, 1 μm. Full size image High-resolution zone plates Spiral zone plates that have previously been used to generate X-rays with orbital angular momentum [26] , [27] were fabricated. A 2 × 2 array of spiral zone plates, each with a square aperture, diameter of 60 μm, smallest outermost zone width of 60 nm, duty cycle of 1:3 and spiral charge of 20 were fabricated. In this case, the adjacent zone plates in the array served as the electron-hole balancing structures. 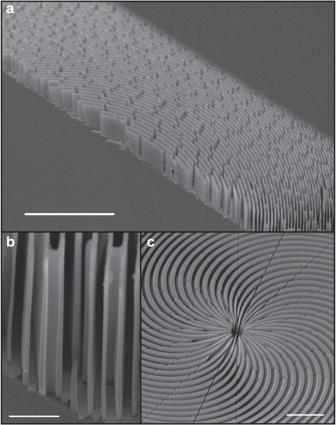Figure 5: High-resolution zone plates. (a) SEM image of a cleaved spiral zone plate from a 2 × 2 array of zone plates. The cross-sectional view shows uniformity in etching depth over a range of feature sizes in the zone plate. Scale bar, 5 μm. (b) Cross-sectional views of some of the small zones in this zone plate. Line widths are ~32 nm and 2.5 μm tall, and the period is 136 nm. Scale bar, 500 nm. (c) A top-down view of the etched zone plate of a charge 20 spiral zone plate. Scale bar, 5 μm. Figure 5a shows a SEM image of the cross-section of this zone plate when mechanically cleaved. Uniformity in the etch depth across the range of feature sizes in the zone plate can be seen. Figure 5b shows zones close to the edge of the zone plate with 32 nm line width and 136 nm period, demonstrating a duty cycle of 1:3. The zones here are 2.5 μm tall creating aspect ratios of ~40:1. Figure 5: High-resolution zone plates. ( a ) SEM image of a cleaved spiral zone plate from a 2 × 2 array of zone plates. The cross-sectional view shows uniformity in etching depth over a range of feature sizes in the zone plate. Scale bar, 5 μm. ( b ) Cross-sectional views of some of the small zones in this zone plate. Line widths are ~32 nm and 2.5 μm tall, and the period is 136 nm. Scale bar, 500 nm. ( c ) A top-down view of the etched zone plate of a charge 20 spiral zone plate. Scale bar, 5 μm. Full size image Platinum metallization and efficiency testing of zone plates For use with hard X-rays, the silicon zone plate mould must be metallized, for example, through atomic layer deposition or electroplating. Electroplating provides high efficiency throughout an entire zone plate area, whereas traditional atomic layer deposition provides the ability to create higher resolution zones with high efficiency, but in a tradeoff of overall zone plate efficiency. A combination of both methods, or variations of these methods, can be envisioned for achieving the benefits of both techniques. In this experiment, Pt atomic layer deposition was performed, and efficiency of the outermost zones was measured at 8.995 keV using the beamline 6.2 transmission X-ray microscope at the Stanford Synchrotron Radiation Lightsource. A silicon zone plate mould was fabricated using V-MACE. A 5-nm layer of Al 2 O 3 followed by a 45-nm layer of Pt were deposited as depicted in Fig. 6a . The final platinum zone plate structure had a 50-nm outermost zone width, 200 μm diameter and 2.1 μm zone thickness. An SEM image of the resulting structure is shown in Fig. 6b . Local zone plate efficiency measurements over a 30-μm diameter outermost zone region resulted in a 20.1% first-order diffraction efficiency. We note that this zone thickness will yield higher efficiencies at energies >10 keV owing to more favourable phase-shifting properties of the Pt zones at higher energies. 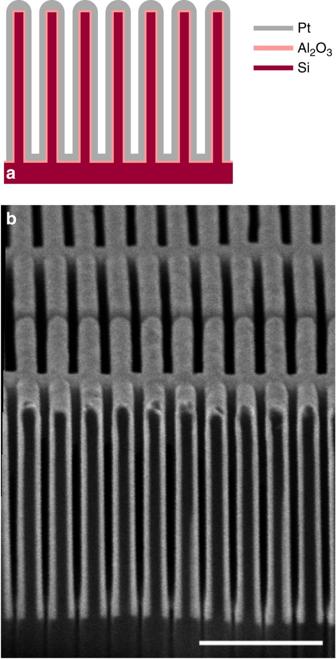Figure 6: Pt metallization for X-ray zone plates. (a) Schematic of Pt atomic layer deposition of Si zone plate structure. The starting Si zone plate mould is shown in red. A 5-nm layer of Al2O3is deposited followed by a 45-nm layer of Pt. The coating is conformal over the entire Si zone plate mould. (b) Cross-sectional SEM image of a focused ion beam sectioned zone plate. The image is taken at a tilt angle of 52 degrees. Scale bar, 1 μm. Figure 6: Pt metallization for X-ray zone plates. ( a ) Schematic of Pt atomic layer deposition of Si zone plate structure. The starting Si zone plate mould is shown in red. A 5-nm layer of Al 2 O 3 is deposited followed by a 45-nm layer of Pt. The coating is conformal over the entire Si zone plate mould. ( b ) Cross-sectional SEM image of a focused ion beam sectioned zone plate. The image is taken at a tilt angle of 52 degrees. Scale bar, 1 μm. Full size image In this paper, we have described how ultra-high aspect ratio etched silicon zone plate moulds were fabricating using V-MACE. Because a zone plate consists of a large range of feature sizes, larger in the centre and smaller in the outermost zones, etch rate variations as a function of zone width needs to be controlled for uniform, vertical etching. We minimize this by using low temperature and low H 2 O 2 concentrations, along with appropriate dimensional variations in the pattern, such as catalyst interconnection density and Si zone buttress density. The low temperature and low H 2 O 2 concentration causes the reduction reaction of H 2 O 2 to become the rate-limiting step in MACE such that the etch rate variation, originally because of different etchant diffusion lengths of different feature sizes, is minimized. This etching method is compatible with other catalyst patterning schemes. In this paper, a liftoff process was used to pattern the metal catalyst, but other methods can be used for patterning including, but not limited to, focused ion beam and reactive ion etching of the metal catalyst. It is important in all cases that the interface between the silicon and the metal catalyst be clean for directional control during the etching. For the work described in this paper, Au catalysts were used. A thin Ti layer was also used, as an adhesion layer for the liftoff process, and later dissolved in the etchant solution. It is well known from the literature that other metal catalysts, such as Ag [28] and Pt [29] , as well as other substrates such as GaAs [30] , can be etched using this method. Therefore, this technique is not limited only to the specific catalyst material and substrate materials used here. This simple fabrication method is suitable for creating optics optimized for the extreme ultraviolet (EUV) to the hard X-ray regime. For the hard X-ray regime, the zone plates can be combined with metallization techniques. Because the metal catalyst sinks to the bottom of the trench after etching, electroplating can be performed for metallization such that a gold zone plate can be made. In addition, atomic layer deposition for coating a variety of different types of materials, optimized for particular wavelengths, can also be performed. For example, Au zone plates with 6 μm thickness could produce up to 35% first-order diffraction efficiency at 25 keV photon energy. Au zone plates with 10 μm thickness could produce close to 40% first-order diffraction efficiency at 50 keV [31] , the maximum efficiency for a binary phase zone plate. In addition, combining two zone plates with different patterns such that a blazed zone plate profile [15] is created through mechanical stacking could further increase the efficiency. For EUV and soft X-rays, etching does not necessarily have to be very deep. As it is currently possible to create nanowires <10 nm wide using conventional MACE, we believe it should be possible to etch similar dimensions for X-ray optics applications through application of V-MACE. In addition, it is also possible to directly use the silicon lens and forgo the metallization or material deposition process for softer X-ray energies. For example, with 50 eV radiation, a silicon zone plate with 280 nm thickness could produce a theoretical first-order efficiency of ~27%. For 700–900 eV wavelength, in the soft X-ray region, a silicon zone plate of 1 μm thickness could produce a theoretical first-order efficiency of ~26–29%. In each of these cases there will be some area loss, resulting in slight lowering of the theoretical efficiency owing to the Si buttress and catalyst anchor density, but overall efficiencies will remain high compared with what is currently available. Volume effects, for example, in the case of vertical outermost zone widths approaching 10 nm and zone thicknesses approaching 1 μm, will cause a reduction in diffraction efficiency unless the zones are tilted or appropriately shaped. In addition, as in the case of hard X-rays, these zone plates can be combined with existing concepts such as stacking to produce shaped, blazed zones, thicker or interleaved structures for increased efficiency. For applications requiring free-standing zone plates, especially important at the low EUV energies, this fabrication process can be performed on commercially available single crystalline Si membranes. In conclusion, we have demonstrated a simple process to fabricate ultra-high aspect ratio, dense features in a complex, non-repetitive nanostructure using vertical directionality controlled MACE, with optimizations of metal catalyst mechanical anchors, hole concentration balancing structures, low temperature etching and low H 2 O 2 concentration for the case of X-ray zone plate optics fabrication. This leads to the capability to create high-efficiency zone plate optics and more general X-ray diffractive optical structures such as coded apertures and collimators for hard X-rays, far beyond what is currently available. The versatility of this ultra-high aspect ratio etching process for nanostructures can also lead to its utilization for a broad array of applications, including sensors and energy-related nanostructured materials, among others. Lithographic process for linear gratings A 60-nm-thick layer of 950 K Polymethyl methacrylate (PMMA) is spin coated onto a P-type, Boron-doped ‹100› CZ Prime silicon wafer with 10–20 Ω cm resistivity (SiliconQuest). The resist layer is then baked at 170 °C for 30 min and patterned with a 100-keV JEOL 6300 electron beam lithography system. The patterned resist was then developed in 1:3 MIBK (methyl isobutyl ketone): IPA (isopropyl alcohol) at 4 °C for 30 s. An oxygen descum etch was performed to remove any residual PMMA. The metal catalyst layer that consists of 2 nm Ti and 15 nm Au is then electron beam evaporated onto the pattern. Liftoff was performed in acetone. The patterned piece and etching solution comprised of 5.3 M HF, 0.25 M H 2 O 2 and 50 M H 2 O are cooled to 10 °C, and a droplet of etchant is placed on top of the pattern. Etching was performed at 10 °C for 40 min and then quenched with a H 2 O rinse. The pattern was dried using nitrogen. Lithographic process for high aspect ratio zone plates A 300-nm-thick layer of ZEP520A is spin coated on a P-type, ‹100› FZ Prime silicon wafer with >10,000 Ω cm resistivity (SiliconQuest). The resist was patterned with a 100-keV JEOL 6300 electron beam lithography system. The patterned resist was then developed in xylenes at 20 °C for 40 s. An oxygen descum etch was performed to remove any residual ZEP520A. The metal catalyst layer, 2 nm Ti and 75 nm Au, was then electron beam evaporated onto the pattern. Liftoff was performed in Remover PG (MicroChem) at 70 °C. The patterned piece and etching solution comprised of 5.3 M HF, 0.25 M H 2 O 2 and 50 M H 2 O were cooled to 6 °C using a cold plate, and a droplet of etchant was placed on top of the pattern. Etching was performed at 6 °C for 90 min and then quenched with a H 2 O rinse. H 2 O was replaced with isopropyl alcohol, and the sample was dried using a critical point dryer (Tousimis). Lithographic process for high-resolution zone plates A 60-nm-thick layer of 950 K PMMA is spin coated onto a P-type, Boron-doped ‹100› CZ Prime silicon wafer with 10–20 Ω cm resistivity (SiliconQuest). The resist layer is then baked at 170 °C for 30 min and patterned with a 100-keV JEOL 6300 electron beam lithography system. The patterned resist was then developed in 1:3 MIBK:IPA at 4 °C for 30 s. An oxygen descum etch was performed to remove any residual PMMA. The metal catalyst layer that consists of 2 nm Ti and 15 nm Au is then electron beam evaporated onto the pattern. Liftoff was performed in acetone. The patterned piece and etching solution comprised of 5.3 M HF, 0.25 M H 2 O 2 and 50 M H 2 O are cooled to 10 °C, and a droplet of etchant is placed on top of the pattern. Etching was performed at 10 °C for 30 min and then quenched with a H 2 O rinse. The pattern was dried using nitrogen. Pt metallization and zone plate efficiency measurement A Si zone plate mould was fabricated using V-MACE. A 5-nm layer of Al 2 O 3 followed by a 45-nm Pt layer was deposited onto the zone plate mould, resulting in a zone plate with 50 nm outermost zone width, 200 μm diameter and 2.1 μm zone thickness. The zone plate was then placed in the transmission X-ray microscope at beamline 6.2 at the Stanford Synchrotron Radiation Lightsource for zone plate efficiency measurements. The energy used for the measurement was 8.995 keV. A 30-μm pinhole diameter was placed behind a portion of the capillary condenser optic of the microscope to restrict the illumination area of the zone plate. In order to obtain the reference intensity, the zone plate was moved out of the way, whereas the radiation still passed through the pinhole and substrate. The intensity of the spot at the CCD was integrated. To obtain the diffracted efficiencies, the zone plate was then placed behind the same illumination area, and the diffracted spots were observed at the CCD. The total radiation of the first-order diffracted spot was integrated, and the first-order diffraction efficiency was calculated by taking the ratio of the radiation in the first-order diffraction spot with the radiation in the reference spot. How to cite this article: Chang, C. and Sakdinawat, A. Ultra-high aspect ratio high-resolution nanofabrication for hard X-ray diffractive optics. Nat. Commun. 5:4243 doi: 10.1038/ncomms5243 (2014).